PIF1 family DNA helicases suppress R-loop mediated genome instability at tRNA genes Saccharomyces cerevisiae encodes two Pif1 family DNA helicases, Pif1 and Rrm3. Rrm3 promotes DNA replication past stable protein complexes at tRNA genes (tDNAs). We identify a new role for the Pif1 helicase: promotion of replication and suppression of DNA damage at tDNAs. Pif1 binds multiple tDNAs, and this binding is higher in rrm3 Δ cells. Accumulation of replication intermediates and DNA damage at tDNAs is higher in pif1 Δ rrm3 Δ than in rrm3 Δ cells. DNA damage at tDNAs in the absence of these helicases is suppressed by destabilizing R-loops while Pif1 and Rrm3 binding to tDNAs is increased upon R-loop stabilization. We propose that Rrm3 and Pif1 promote genome stability at tDNAs by displacing the stable multi-protein transcription complex and by removing R-loops. Thus, we identify tDNAs as a new source of R-loop-mediated DNA damage. Given their large number and high transcription rate, tDNAs may be a potent source of genome instability. During each S-phase, the replication machinery encounters multiple classes of naturally occurring structures that impede fork progression. These structures include stable protein complexes, highly transcribed genes and stable DNA secondary structures [1] . Paused replication forks are particularly susceptible to breakage owing to the single-stranded DNA at the fork. Repair of these double strand breaks (DSBs) can promote recombination between direct repeats or lead to complex genetic events (gross chromosomal rearrangements, GCRs), which occur in many human cancers [2] . Pif1 family DNA helicases are present in virtually all eukaryotes. While most eukaryotes, including humans, encode a single Pif1 family DNA helicase, Saccharomyces cerevisiae encodes two, Rrm3 and Pif1 (ref. 3). Although Pif1 and Rrm3 often affect the same substrates, they do not necessarily act in the same way [3] ; e.g., Pif1 inhibits telomerase, while Rrm3 promotes semiconservative replication of telomeric DNA. In addition to inhibiting telomerase, Pif1 (but not Rrm3) is required for stable maintenance of mitochondrial DNA, Okazaki fragment maturation and break induced replication [4] . Pif1 also promotes replication and suppresses DNA damage at sequences that can form G-quadruplex structures in vitro [4] . Rrm3 is best known for promoting fork progression at stable protein–DNA complexes [5] , [6] . Rrm3 moves with the replication fork [7] , while Pif1 is probably recruited to its sites of action [8] (C.-F.C., S.P., T.J.P. and V.A.Z., manuscript in preparation). Understanding the mechanism(s) by which Pif1 family helicases affect genome integrity is relevant to human disease, as mutation of mammalian PIF1 family helicases is associated with increased risk of breast cancer [9] and mitochondrial myopathies [10] . From yeasts to humans, stable protein–DNA complexes and R-loops are natural replication impediments [11] . Both of these structures occur at tDNAs. In S. cerevisiae , when replication and transcription move in opposite directions through a tDNA, forks slow even in wild type (WT) cells [12] . Rrm3 promotes fork progression at RNA Polymerase (Pol) III transcribed genes, such that in its absence, these genes become among the most potent naturally occurring impediments to fork progression [5] , [13] . Mutation of the tDNA promoter so that it is unable to assemble the transcription initiation complex eliminates pausing at the tDNA in both WT and rrm3 Δ cells [5] . However, a more than 3-fold increase in the size of the transcribed tDNA does not increase the size or extent of replication pausing at the gene. These data suggest that Rrm3 acts by promoting fork movement past the particularly stable, multiprotein pre-initiation complex that is rapidly recycled such that many tDNAs are almost always pre-initiation complex associated [14] , [15] . Using S. cerevisiae and genome-wide approaches, several laboratories have detected R-loops not only at highly transcribed RNA Pol II genes, but also at tDNAs [16] , [17] , [18] . From yeasts to humans, R-loops cause DNA damage at RNA Pol II transcribed genes [19] , [20] , [21] , [22] , but, to our knowledge, R-loop-mediated DNA damage has not been detected at RNA Pol III-transcribed genes in any organism. There are ∼ 1,400 discrete sites in the S. cerevisiae genome that depend on Rrm3 for timely replication, including ∼ 425 RNA Pol III transcribed genes, such as the 274 tDNAs, ∼ 150 5S rRNA genes and other small RNAs (e.g., SCR1 and RPR1 ) [5] , [13] , [23] . Although rrm3 Δ cells are viable, they require DNA damage checkpoints and fork restart activities to survive [5] , [24] , [25] . Given the importance of Rrm3 for tDNA and 5S gene replication, we reasoned that there might be another DNA helicase that acts as a backup for Rrm3 at these hard-to-replicate sites. Indeed, rrm3 Δ cells are not viable in the absence of at least two DNA helicases, Srs2 and Sgs1, but both of these helicases act after DNA replication, as the lethality in the double mutants ( srs2Δ rrm3 Δ and sgs1 Δ rrm3 Δ) is suppressed by deleting RAD51 (refs 25,26). Although pif1 Δ rrm3 Δ cells are viable, they grow very slowly. Therefore, we hypothesized that Pif1 might act as a backup for Rrm3 during replication of tDNAs. Here we show that tDNAs not only slow DNA replication, they also cause DNA damage, and this damage is due to R-loops. Pif1 binds robustly to multiple tDNAs. Fork pausing and R-loop-mediated DNA damage are both exacerbated in pif1-m2 rrm3 Δ or pif1 Δ rrm3 Δ cells, compared to single mutants ( pif1-m2, pif1 Δ or rrm3 Δ). Thus, the Pif1 family DNA helicases, Rrm3 and Pif1, act together to promote replication and suppress R-loop mediated DNA damage at tDNAs. Pif1 and Rrm3 bind to multiple tDNAs As a first step to determine if Pif1 acts at tDNAs, we used chromatin-immunoprecipitation and quantitative PCR (ChIP-qPCR) to ask if Pif1 bound three tDNAs whose replication is Rrm3-sensitive [5] (see also Fig. 2a,b and Supplementary Fig. 2 ): tDNA ala ( tA(AGC)F ), tDNA tyr ( tY(GUA)F1 ) and tDNA gly ( tG(GCC)J2 ). For both Pif1 and Rrm3, their binding to tDNAs (ChIP/input) was normalized to YBL028C , a control sequence with low binding to both helicases. Pif1 binding to the three tDNAs was highly significant (P ⩽ 0.0009) compared to the control sequence ( Fig. 1a ). Moreover, the binding of Pif1 to the three tDNAs was significantly higher in rrm3 Δ than in WT cells (P ⩽ 0.007). This increased Pif1 binding in rrm3 Δ cells was not due to increased Pif1 abundance ( Fig. 1c ). 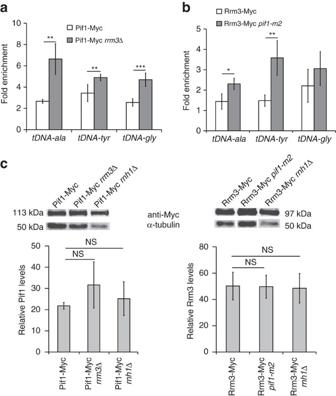Figure 1: Pif1 and Rrm3 bind tDNAs. Enrichment of Pif1 (ChIP/input) or Rrm3 (ChIP/input) at tDNAs was normalized to helicase enrichment atYBL028C, a site that has low binding to both helicases. (a) Fold enrichment ([ChIP/input]tDNA/[ChIP/input]YBL028C) of Pif1-Myc in asynchronous wild-type (WT) and inrrm3Δ cells attDNAalaHO,tDNAtyrHO andtDNAglyHO. (b) Fold enrichment of Rrm3-Myc in asynchronous WT andpif1-m2cells attDNAalaHO,tDNAtyrHO andtDNAglyHO. Full blots are shown inSupplementary Fig. 7. (c) Western blot (top) and its quantification (bottom) showing Pif1 or Rrm3 expression levels in WT,rrm3Δ,pif1-m2andrnh1Δ cells. All quantification was normalized to the loading control, α-tubulin. The difference in Pif1 abundance between WT andrrm3Δ orrnh1Δ cells was not significant (NS) (P>0.05). Similarly, Rrm3 abundance was the same between WT andpif1-m2orrnh1Δ cells. Error bars are±s.d. for at least three independent experiments per strain.P-values here and elsewhere were obtained using unpaired two-tailed Student’st-test. Here and in subsequent figures, * indicatesP<0.05, ** indicatesP⩽0.009, and *** indicatesP⩽0.0009. Figure 1: Pif1 and Rrm3 bind tDNAs. Enrichment of Pif1 (ChIP/input) or Rrm3 (ChIP/input) at tDNAs was normalized to helicase enrichment at YBL028C , a site that has low binding to both helicases. ( a ) Fold enrichment ([ChIP/input] tDNA /[ChIP/input] YBL028C ) of Pif1-Myc in asynchronous wild-type (WT) and in rrm3 Δ cells at tDNA ala HO, tDNA tyr HO and tDNA gly HO. ( b ) Fold enrichment of Rrm3-Myc in asynchronous WT and pif1-m2 cells at tDNA ala HO, tDNA tyr HO and tDNA gly HO. Full blots are shown in Supplementary Fig. 7 . ( c ) Western blot (top) and its quantification (bottom) showing Pif1 or Rrm3 expression levels in WT, rrm3 Δ, pif1-m2 and rnh1 Δ cells. All quantification was normalized to the loading control, α-tubulin. The difference in Pif1 abundance between WT and rrm3 Δ or rnh1 Δ cells was not significant (NS) ( P >0.05). Similarly, Rrm3 abundance was the same between WT and pif1-m2 or rnh1 Δ cells. Error bars are±s.d. for at least three independent experiments per strain. P -values here and elsewhere were obtained using unpaired two-tailed Student’s t -test. Here and in subsequent figures, * indicates P <0.05, ** indicates P ⩽ 0.009, and *** indicates P ⩽ 0.0009. 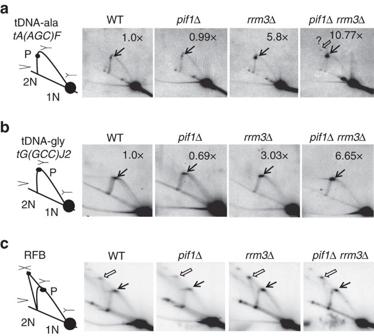Figure 2: Forks stall but do not arrest at tDNAs in the absence of Pif1 family DNA helicases. DNA from asynchronous WT,pif1Δ,rrm3Δ orpif1Δrrm3Δ cells was digested with restriction enzymes and analysed by two-dimensional (2D) gel electrophoresis and Southern hybridization. (a–c) Schematics of the results from 2D gel analysis for each region are shown to the left of the Southern blots of 2D gels: 1N marks the position of non-replicating linear fragments; 2N is position of almost fully replicated 1N fragments right before sister chromatids separate; P, replication pause; X, converged forks. Southern blots were hybridized using32P-labelled probes to detect the following regions (seeSupplementary Table 10for primers for probes): (a)tDNAalaHO (BglII), (b)tDNAglyHO (EcoRI) and (c) rDNA (BglII fragment containing RFB). Black arrows indicate sites of fork pausing and open arrows indicate sites of converged forks. Ina, there is a faint signal at tDNAalainpif1Δrrm3Δ cells that might be due to converged forks; this signal is marked with an open arrow and a question mark. Ina,b, the signal at the pause was quantified (seeSupplementary Fig. 1for details) and normalized to the pause signal in WT cells to obtain the relative fold change (top right corner of each Southern blot). The average fold difference of 2D gels from two independent biological replicates fortDNAalais shown inSupplementary Fig. 1.cis a 2D gel from the same DNA preparation used inbthat was hybridized with an rDNA probe to visualize forks converged at the RFB. Full size image Figure 2: Forks stall but do not arrest at tDNAs in the absence of Pif1 family DNA helicases. DNA from asynchronous WT, pif1 Δ, rrm3 Δ or pif1 Δ rrm3 Δ cells was digested with restriction enzymes and analysed by two-dimensional (2D) gel electrophoresis and Southern hybridization. ( a – c ) Schematics of the results from 2D gel analysis for each region are shown to the left of the Southern blots of 2D gels: 1N marks the position of non-replicating linear fragments; 2N is position of almost fully replicated 1N fragments right before sister chromatids separate; P, replication pause; X, converged forks. Southern blots were hybridized using 32 P-labelled probes to detect the following regions (see Supplementary Table 10 for primers for probes): ( a ) tDNA ala HO (BglII), ( b ) tDNA gly HO (EcoRI) and ( c ) rDNA (BglII fragment containing RFB). Black arrows indicate sites of fork pausing and open arrows indicate sites of converged forks. In a , there is a faint signal at tDNA ala in pif1 Δ rrm3 Δ cells that might be due to converged forks; this signal is marked with an open arrow and a question mark. In a , b , the signal at the pause was quantified (see Supplementary Fig. 1 for details) and normalized to the pause signal in WT cells to obtain the relative fold change (top right corner of each Southern blot). The average fold difference of 2D gels from two independent biological replicates for tDNA ala is shown in Supplementary Fig. 1 . c is a 2D gel from the same DNA preparation used in b that was hybridized with an rDNA probe to visualize forks converged at the RFB. Full size image Because Rrm3 moves with the replisome, all nuclear sequences are Rrm3-associated at their time of replication [7] . Thus, it was not unexpected that Rrm3 binding to the three tDNAs was only modestly (1.5- to 2-fold) higher than to the control sequence ( Fig. 1b ). However, in pif1-m2 cells, which are deficient in nuclear but not mitochondrial Pif1 (ref. 27), Rrm3 binding to two of the three tDNAs was significantly higher than in WT cells ( P ⩽ 0.01). This higher binding was not due to increased Rrm3 abundance in pif1-m2 cells ( Fig. 1c ). Together, these binding patterns suggest that Pif1, like Rrm3, acts at tDNAs and that the action of both helicases at tDNAs may be more important in the absence of the other helicase. Pif1 is important for tDNA replication in rrm3 Δ cells The extent to which a tDNA impedes fork progression is dependent on the direction of replication through the gene. When replication and transcription move through a tDNA in the same direction (CD, co-directional), the tDNA has less impact on fork progression than when replication and transcription move in opposite directions (HO, head on orientation) [5] , [12] . The three tDNAs examined by ChIP-qPCR for Pif1 and Rrm3 binding ( Fig. 1a,b ) are all in the HO orientation [5] . In previous work, we used two-dimensional gel (2D gels) electrophoresis [5] and genome-wide analyses [13] to show that fork progression is slowed at many, and perhaps all, tDNAs in the absence of Rrm3, and this effect occurred for tDNAs in both HO and CD orientations. Here we used 2D gels to determine if Pif1 affects replication at the three tDNAs analysed by ChIP-qPCR ( Fig. 1a,b ). Replication of each tDNA was examined at the gene’s native chromosomal locus ( Fig. 2a,b and Supplementary Fig. 1, 2 ). As expected, pausing at tDNAs was increased in rrm3 Δ cells compared to WT cells ( ∼ 6-fold at tDNA ala HO and ∼ 3-fold at tDNA gly HO). The extent of pausing at both tDNAs was similar in pif1 Δ and WT cells. However, in pif1 Δ rrm3 Δ cells, pausing at both tDNAs was significantly higher ( ∼ 11-fold at tDNA ala HO and ∼ 7-fold at tDNA gly HO) than in WT, pif1 Δ or rrm3 Δ cells. Similar results were seen for tDNA tyr HO ( Supplementary Fig. 2 ). The replication pattern was comparable for tDNA ala HO when the partial loss of function allele pif1-m2 was used in place of pif1 Δ ( Supplementary Fig. 4b ). These data demonstrate that Pif1 promotes replication through tDNAs in rrm3 Δ cells. Recently, it was argued that forks do not pause but rather terminally arrest at tDNAs in rrm3 Δ cells, and this terminal arrest is increased in cells lacking both Pif1 family helicases [28] . Terminal replication arrest generates converged replication forks at the site of the arrest, as seen by 2D gels at the replication fork barrier (RFB) in ribosomal DNA (rDNA) [29] . However, we saw no evidence for the X structures in rrm3 Δ cells that are characteristic of converged forks at any of the eight tDNAs examined either here or in published 2D gels [12] (see also Fig. 2a,b and Supplementary Figs 2c, 3, 4b ). One explanation for the failure to detect converged forks at tDNAs is that these structures were lost during DNA extraction or 2D gel analysis. To test this possibility, the same DNA preparation used to examine replication of tDNA gly HO ( Fig. 2b ) was tested subsequently for 2D gel analysis of rDNA replication ( Fig. 2c ). We chose an exposure where the signal in the 1N spot of unreplicated DNA molecules was lower in rDNA than in tDNA to ensure that the exposure for the tDNA was sufficient to detect converged forks at a single copy gene. The well-documented arrest and converged forks at the RFB were readily detectable in mutant and WT strains. Likewise, reprobing the Southern blots of tDNA ala HO 2D gels with the rDNA probe detected converged forks at the RFB ( Supplementary Fig. 3 ). Of course, even without terminal fork arrest, converged forks could occur transiently at tDNAs if moving forks from flanking origins meet at the tDNA. Fork convergence is more likely if the tDNA is about equi-distant from the two flanking origins. Convergence of moving forks at tDNA gly is unlikely as this gene is predominately replicated by ARS1018 , an early, efficient origin that is only 8.6 kb from the gene on its telomere-proximal side [30] , [31] , [32] . The nearest origin to tDNA gly on the centromere-proximal side is ARS1017, an early origin that is located 72 kb away. However, at tDNA ala , the gene is 5.4 and 11.4 kb from the flanking origins ( ARS607 and ARS608 , respectively) [31] , [32] , [33] . Thus, forks could converge occasionally at tDNA ala if the more distal origin fires before the closer origin in some S phases. Indeed, while we saw no converged forks at tDNA ala in WT, pif1 Δ, or rrm3 Δ cells ( Fig. 2a ; Supplementary Fig. 3 ), in pif1 Δ rrm3 Δ cells, there was an extremely weak but reproducible signal in the 2D gel that could be explained by forks converged at the tDNA (marked by open arrow and a question mark in Fig. 2a and Supplementary Fig. 3 ). We conclude from analysing replication of multiple tDNAs in their native chromosomal loci by 2D gels that fork arrest at tDNAs is very rare, not only in WT cells but also in the absence of Pif1 and/or Rrm3. Fork arrest at tDNAs is much rarer than in rDNA, where it is estimated to occur in fewer than 20% of the repeats [29] . Pif1 and Rrm3 suppress direct repeat recombination at tDNAs To determine if fork pausing at tDNAs causes DNA damage, we used two different genetic assays where the read-out is sensitive to the occurrence of DSBs. The first assay monitors recombination between direct repeats (DR) of portions of the ADE2 gene, which are separated by a region containing URA3. In this assay, recombination generates FOA-resistant Ade2 + cells, and the occurrence of cells of this genotype is increased by a DSB between the repeats [8] , [34] ( Fig. 3a ). By 2D gel analysis, tDNA ala HO caused fork pausing when inserted into the DR substrate, just as it did at its endogenous locus ( Supplementary Fig. 4 ). 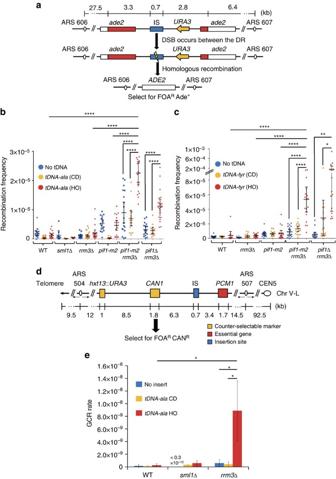Figure 3: Pif1 family DNA helicases suppress DSB-induced recombination at tDNAs. (a) Schematic of the direct repeat (DR) recombination construct generated on the right arm of chromosome VI. Blue box indicates site of tDNA insertions (IS) wheretDNAalaortDNAtyrwas inserted in head-on (HO) or co-directional (CD) orientation. Different parts ofADE2(red and white bars), neither of which is sufficient to generate Ade+cells, are separated by∼5 kb containingURA3.A double-strand break (DSB) between theade2segments initiates recombination between the two partial copies ofADE2, which generates FOARAde+cells. (b,c) Recombination frequencies in cells with no insert or containingtDNAala(b) ortDNAtyr(c) in HO or CD orientations were determined by dividing the number of FOARAde+cells by the number of viable cells that grew on non-selective plates. The means of the recombination frequencies with 95% confidence interval were calculated from at least three independent technical and biological replicates per strain. The mean±s.d. is also provided inSupplementary Tables 5 and 7. (d) Schematic of the left arm of chromosome V (Chr V-L) in gross chromosomal rearrangement (GCR) strains.tDNAalaHO ortDNAalaCD was inserted at insertion site (IS in blue box) in GCR strains. Genes within the 45 kb test interval are non-essential;PCM1(red box) is an essential gene, the most distal essential gene on ChrV-L. A DSB that occurs upstream of the two marker genes,URA3andCAN1(yellow boxes), initiates GCR events, which are monitored by selecting for FOARCanRcells. (e) GCR rates with or withouttDNAalaCD or HO inserts were calculated using FALCOR and MMS maximum likelihood method64. Means and standard deviations of GCR rates were obtained from at least three technical replicates of two different isolates per strain. Here, * indicatesP<0.05, ** indicatesP⩽0.009, and **** indicatesP<0.0001. Figure 3: Pif1 family DNA helicases suppress DSB-induced recombination at tDNAs. ( a ) Schematic of the direct repeat (DR) recombination construct generated on the right arm of chromosome VI. Blue box indicates site of tDNA insertions (IS) where tDNA ala or tDNA tyr was inserted in head-on (HO) or co-directional (CD) orientation. Different parts of ADE2 (red and white bars), neither of which is sufficient to generate Ade + cells, are separated by ∼ 5 kb containing URA3. A double-strand break (DSB) between the ade2 segments initiates recombination between the two partial copies of ADE2 , which generates FOA R Ade + cells. ( b , c ) Recombination frequencies in cells with no insert or containing tDNA ala ( b ) or tDNA tyr ( c ) in HO or CD orientations were determined by dividing the number of FOA R Ade + cells by the number of viable cells that grew on non-selective plates. The means of the recombination frequencies with 95% confidence interval were calculated from at least three independent technical and biological replicates per strain. The mean±s.d. is also provided in Supplementary Tables 5 and 7 . ( d ) Schematic of the left arm of chromosome V (Chr V-L) in gross chromosomal rearrangement (GCR) strains. tDNA ala HO or tDNA ala CD was inserted at insertion site (IS in blue box) in GCR strains. Genes within the 45 kb test interval are non-essential; PCM1 (red box) is an essential gene, the most distal essential gene on ChrV-L. A DSB that occurs upstream of the two marker genes, URA3 and CAN1 (yellow boxes), initiates GCR events, which are monitored by selecting for FOA R Can R cells. ( e ) GCR rates with or without tDNA ala CD or HO inserts were calculated using FALCOR and MMS maximum likelihood method [64] . Means and standard deviations of GCR rates were obtained from at least three technical replicates of two different isolates per strain. Here, * indicates P <0.05, ** indicates P ⩽ 0.009, and **** indicates P <0.0001. Full size image In both genetic assays, we determine if tDNAs affect recombination by comparing the number of recombination events within a strain with or without (‘no insert’) a tDNA in the test interval. Insertion of tDNA ala HO ( Fig. 3b ) or tDNA tyr HO ( Fig. 3c ) in the DR assay did not cause a significant increase in recombination in rrm3 Δ cells compared to the no insert control ( Table 1 ). Similarly, in a pif1-m2 strain, DR recombination was not increased significantly by the presence of either tDNA ala or tDNA tyr (CD and HO for both). However, the recombination frequency in pif1-m2 rrm3 Δ cells was significantly higher in the presence of tDNA ala HO ( ∼ 2.5-fold) and tDNA tyr HO ( ∼ 6-fold) compared to no tDNA, tDNA ala CD or tDNA tyr CD ( Table 1 ). Table 1 Fold increase of DR recombination frequency relative to no tDNA insert. Full size table Because pif1-m2 is not a null allele [27] , the DR recombination experiment was also carried out in pif1 Δ and pif1 Δ rrm3 Δ cells ( Fig. 3b,c and Supplementary Fig. 5b,c ). Although mitochondrial deficiency increased the background level of DR recombination ( Supplementary Fig. 5a ), neither tDNA ala HO nor tDNA tyr HO affected the frequency of DR recombination in pif1 Δ cells compared to the no insert control ( Supplementary Fig. 5b,c ). However, insertion of either tDNA caused a highly significant increase in DR recombination in pif1 Δ rrm3 Δ cells (3.6-fold for tDNA ala HO and 52.6-fold for tDNA tyr HO) ( Fig. 3b,c and Table 1 ). This increase in pif1 Δ rrm3 Δ cells was higher than in pif1-m2 rrm3 Δ cells. This result is consistent with pif1-m2 being a partial loss of function allele. Taken together, these data indicate that Rrm3 and Pif1 act synergistically to suppress DNA damage, as inferred from the frequency of DR recombination at tDNAs. tDNAs increase gross chromosomal events in rrm3 Δ cells In rrm3 Δ cells, DR recombination was increased at tDNA ala HO (1.9-fold) and tDNA tyr HO (3.2-fold), but neither increase was significant ( Fig. 3b,c and Table 1 ). Because fork pausing increases dramatically at tDNAs in rrm3 Δ cells [5] (see also Fig. 2a,b ), we decided to examine the effects of tDNAs on chromosome breakage in a GCR assay [35] , which is more sensitive than the DR assay. This assay detects complex genetic rearrangements within the non-essential ∼ 45 kb terminal portion of the left arm of chromosome V ( Fig. 3d ). (This assay is not well suited to study damage in pif1-m2 or pif1 Δ cells, as most DSBs in these backgrounds are repaired by telomere addition (TA), not recombination [36] ; because rrm3 Δ partially suppresses the TA phenotype of pif1 Δ cells, GCR events in the double mutant arise by both TA and recombination [37] .) As reported earlier [24] , in the parent strain (no tDNA in the test interval), rrm3 Δ cells had a GCR rate similar to WT cells ( Fig. 3e and Supplementary Table 1 ). In WT cells, insertion of tDNA ala HO or tDNA ala CD did not increase the GCR rate significantly ( Fig. 3e and Table 2 ). In contrast, the GCR rate in rrm3 Δ cells was 15-fold higher with tDNA ala HO than in the no insert control or in the tDNA ala CD. dNTP pools are increased in the absence of Rrm3 (ref. 38). To rule out the possibility that the increase of GCR rate in rrm3 Δ cells was due to higher dNTP pools, GCR rates were also determined in a sml1 Δ strain ( SML1 encodes an inhibitor of ribonucleotide reductase [39] ). There was no increase in GCR rate in sml1 Δ cells with tDNA ala HO or tDNA ala CD ( Fig. 3e ). Thus, the tDNA-dependent increase in GCR rate in rrm3 Δ cells cannot be explained by increased dNTP pools. Table 2 Fold increase of GCR rate relative to no tDNA insert. Full size table R-loops cause DNA damage at tDNAs Genome-wide studies in S. cerevisiae detect R-loops at RNA Pol III transcribed genes, including tDNAs [16] , [17] , [18] . However, to our knowledge, the effects of R-loops at tDNAs on genome integrity have not been examined in any organism. Like R-loops at RNA Pol II transcribed genes [40] , [41] , R-loops at tDNAs are increased in RNaseH-depleted cells [16] , [17] , [18] . Thus, we determined if the tDNA-associated DNA damage seen in rrm3 Δ and pif1-m2 rrm3 Δ cells was due to R-loops. This hypothesis is appealing as Pif1 unwinds RNA-DNA hybrids in vitro much more efficiently than duplex DNA [42] , [43] . First we asked if Pif1 and/or Rrm3 binding to the three tDNAs studied in other experiments in this paper was sensitive to the presence of R-loops by performing ChIP-qPCR in rnh1 Δ cells, which lack RNaseH1. S. cerevisiae encodes a second RNaseH, Rnh201. Like Rnh1, Rnh201 removes R-loops, but it also removes ribonucleotides mis-incorporated during DNA replication [44] , and, therefore, its deletion increases genome instability [45] , [46] . As deleting RNH1 does not cause genome instability [46] , we used Rnh1 deletion or Rnh1 overexpression for all R-loop assays. Because Rnh201 is present in rnh1 Δ cells and able to destabilize R-loops, data in rnh1 Δ cells underestimate the impact of R-loops on DNA damage at tDNAs. Pif1 and Rrm3 association with all three tDNAs were significantly higher in the absence of Rnh1 ( Fig. 4a,b ). The abundance of Pif1 and Rrm3 was not affected by the absence of Rnh1 ( Fig. 1c ). These findings suggest that the functions of both Pif1 family helicases at tDNAs may be more important in cells with stabilized R-loops, as occurs in rnh1 Δ cells. 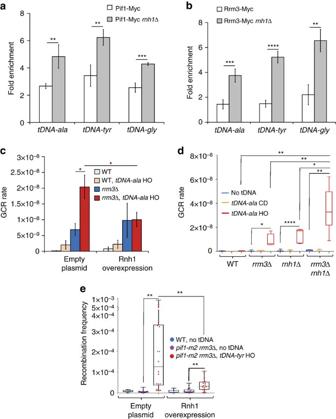Figure 4: tDNA-mediated damage in cells lacking Pif1 family helicases is due to R-loops. In each panel, data are from at least three independent technical and biological replicates per strain. (a,b) ChIP-qPCR analyses of Pif1-Myc and Rrm3-Myc binding totDNAalaHO,tDNAtyrHO andtDNAglyHO in asynchronous WT andrnh1Δ cells. Fold enrichment was calculated as inFig. 1a,b. Error bars are ±s.d. for at least three independent experiments per strain.P-values here and elsewhere were obtained using unpaired two-tailed Student'st-test. (c) Means of GCR rates±s.d. in indicated strains. Cells carry either an empty or Rnh1 overexpression plasmid. (d) The distributions of events determined in the GCR assays in the indicated strains with or withouttDNAalainserts are presented in box-and-whisker plots. The means of the GCR rates with 95% confidence interval were calculated from at least three independent technical and biological replicates per strain. Means of GCR rates±s.d. are also provided inSupplementary Table 1. (e) The recombination frequencies in the indicated strains with empty or Rnh1 overexpression plasmid are presented as box-and-whisker plots. The means of the recombination frequencies with 95% confidence interval were calculated from at least three independent technical and biological replicates per strain. Means of recombination frequencies±s.d are presented inSupplementary Table 7. Here, * indicatesP<0.05, ** indicatesP⩽0.009, *** indicatesP⩽0.0009, and **** indicatesP<0.0001. Figure 4: tDNA-mediated damage in cells lacking Pif1 family helicases is due to R-loops. In each panel, data are from at least three independent technical and biological replicates per strain. ( a , b ) ChIP-qPCR analyses of Pif1-Myc and Rrm3-Myc binding to tDNA ala HO, tDNA tyr HO and tDNA gly HO in asynchronous WT and rnh1 Δ cells. Fold enrichment was calculated as in Fig. 1a,b . Error bars are ±s.d. for at least three independent experiments per strain. P -values here and elsewhere were obtained using unpaired two-tailed Student's t -test. ( c ) Means of GCR rates±s.d. in indicated strains. Cells carry either an empty or Rnh1 overexpression plasmid. ( d ) The distributions of events determined in the GCR assays in the indicated strains with or without tDNA ala inserts are presented in box-and-whisker plots. The means of the GCR rates with 95% confidence interval were calculated from at least three independent technical and biological replicates per strain. Means of GCR rates±s.d. are also provided in Supplementary Table 1 . ( e ) The recombination frequencies in the indicated strains with empty or Rnh1 overexpression plasmid are presented as box-and-whisker plots. The means of the recombination frequencies with 95% confidence interval were calculated from at least three independent technical and biological replicates per strain. Means of recombination frequencies±s.d are presented in Supplementary Table 7 . Here, * indicates P <0.05, ** indicates P ⩽ 0.009, *** indicates P ⩽ 0.0009, and **** indicates P <0.0001. Full size image To confirm the interpretation that tDNA-associated DNA damage in the GCR assay in rrm3 Δ cells was due to R-loops, we used a plasmid containing a galactose-inducible RNH1 gene [47] . The high GCR rate observed in rrm3 Δ cells containing tDNA ala HO was significantly reduced by overexpression of Rnh1 (p<0.05) ( Fig. 4c and Table 3 ). Indeed, when Rnh1 was overexpressed, the GCR rate was identical in rrm3 Δ cells with and without tDNA ala HO. Likewise, deleting RNH1 , which stabilizes R-loops [16] , [17] , [18] , significantly increased tDNA-mediated GCR events ( P <0.0001) ( Fig. 4d and Table 2 ). Table 3 Fold increase of GCR rate ( rrm3 Δ) or DR recombination frequency ( pif1-m2 rrm3 Δ) relative to no tDNA insert with or without Rnh1 overexpression. Full size table We also determined the effects of Rnh1 overexpression on DR recombination in pif1-m2 rrm3 Δ cells containing tDNA tyr HO ( Fig. 4e and Table 3 ). As with the GCR rate in rrm3 Δ cells, the frequency of DR recombination in pif1-m2 rrm3 Δ cells was significantly reduced by Rnh1 overexpression ( P =0.004) ( Fig. 4e and Table 3 ). Taken together, these data make a compelling argument that DNA damage at tDNAs is due at least in part to R-loops. Previous studies found that Pif1 and Rrm3 have non-overlapping functions at telomeres [37] , rDNA [23] , mitochondrial DNA [48] and during break induced replication [49] . However, at G-quadruplex (G4) structures, the two helicases act similarly: Pif1 promotes replication and suppresses DNA damage at G4 forming sequences [8] , [50] , [51] , [52] , as does Rrm3 in cells lacking Pif1 (ref. 53). Here we show that Pif1 is a backup for Rrm3 during replication of tDNAs. First, like Rrm3, Pif1 bound robustly to three of three tDNAs-HO, and this binding was higher in rrm3 Δ cells ( Fig. 1a ). Second, by 2D gel analysis, pausing at the same three tDNAs was higher in pif1 Δ rrm3 Δ (or pif1-m2 rrm3 Δ) than in rrm3 Δ cells ( Fig. 2a,b and Supplementary Fig. 2 ). Third, DNA damage was higher in pif1 Δ rrm3 Δ (or pif1-m2 rrm3 Δ) cells than in single mutants at two of two tDNAs-HO ( Fig. 3b,c ). Whereas 2D gels monitor fork progression, the genetic assays determine a possible downstream effect of pausing, DNA damage. Yeast tDNAs form R-loops [16] , [17] , [18] , and R-loops cause DNA damage at RNA Pol II genes [20] , [21] , [22] . To assess if R-loops cause damage at tDNAs, we determined the effects of different levels of RNaseH1 on tDNA-associated damage ( Fig. 4c–e ). In rrm3 Δ cells, DNA damage at tDNA ala HO was reduced to the same level as at the ‘no insert’ control by overexpressing Rnh1, which removes R-loops ( Fig. 4c ) and increased in rnh1 Δ cells, which stabilizes R-loops ( Fig. 4d ). Likewise, the high level of DNA damage at tDNA tyr HO in pif1-m2 rrm3 Δ cells was reduced by Rnh1 overexpression ( Fig. 4e ). We conclude that R-loops at tDNA ala HO and tDNA tyr HO are responsible, at least in part, for tDNA-induced DNA damage, and this damage is suppressed by Pif1 family helicases. In vitro Pif1 has the unusual property of being particularly active at unwinding RNA–DNA hybrids [42] , [43] . It also displaces proteins from DNA [54] . Both of these activities are relevant to fork progression at tDNAs. Because Rrm3 is difficult to purify, its in vitro properties are not well characterized. However, its ability to suppress R-loop caused DNA damage at tDNAs ( Fig. 4c,d ) suggests that it is proficient at unwinding RNA–DNA hybrids in vivo . At several of its in vivo targets, such as tDNAs, the RFB, inactive origins and transcriptional silencers, Rrm3 promotes DNA replication by countering the inhibitory effects of stable protein complexes on fork progression [5] , [6] . Given its biochemical activities, Pif1 may back up Rrm3 not only by unwinding R-loops but also by displacing proteins, and these actions may occur both at tDNAs and other Rrm3 targets. The effects of Pif1 family helicases on tDNA replication was recently examined genome-wide using sequencing of Okazaki fragments generated in DNA ligase I-deficient cells [28] . That study identified Pif1 is a backup for Rrm3 during tDNA replication. That study did not determine if tDNA pausing causes DNA damage, but observed that R-loops are not responsible for replication defects at tDNAs. In combination with our data, these results suggest that replication pausing and DNA damage at tDNAs are separable events. While sharing some overlapping conclusions, our interpretations differ from those of Osmundson et al . [28] regarding the nature of the replication defect at tDNAs. The patterns of Okazaki fragment abundance suggest that replication forks terminally arrest at tDNAs, leading the authors to argue that tDNAs are ‘point terminators’ [28] . The authors sought to validate this interpretation using 2D gels. To this end, they examined replication of a single tDNA on a circular plasmid. Although structures consistent with converged forks at the tDNA are detected, the use of a circular plasmid makes it impossible to determine if they arise from pausing or arrest at the tDNA [28] . In contrast, we examined replication of multiple tDNAs at their native chromosomal locations and saw no convincing evidence for converged forks, even though converged forks in rDNA were readily detected in the same DNA samples ( Fig. 2c and Supplementary Fig. 3 ). Likewise, in the original paper describing replication at tDNAs, the authors concluded that forks pause, rather than arrest, at tDNAs because they did not detect converged forks in their 2D gels [12] . The discrepancy in results between the two labs is probably due to the different methodologies. For example, analyses of the distribution of Okazaki fragments does not detect replication defects at several classes of well-documented pause sites, such as centromeres and highly transcribed RNA Pol II genes [28] . We conclude that forks pause, rather than arrest, at tDNAs, even in pif1 Δ rrm3 Δ cells where pausing was particularly robust. Of course, fork arrest may occur infrequently at many tDNAs, especially if the tDNA is similarly distant from flanking origins. Of the many tDNAs examined by 2D gels by us and others, the only hint of forks converging at a chromosomal tDNA gene was at tDNA ala , and even here the hint of converged forks was weak and only detected in pif1 Δ rrm3 Δ cells ( Fig. 2 and Supplementary Fig. 3 ). We propose a model where Rrm3 is usually responsible for dissociating the stable pre-initiation transcription complex and removing R-loops at tDNAs. Because Rrm3 moves with the replisome [7] , we propose that it acts at the time of tDNA replication ( Fig. 5 ). Based on our ChIP, genetic and 2D gel data and Pif1’s known biochemical activities, we propose that Pif1 has a back-up role in removing R-loops and proteins from tDNAs. Because fork pausing [5] , [12] and DNA damage ( Fig. 3b,c ) were much higher at tDNAs-HO where transcription and replication collide than at tDNAs-CD, we think that most R-loop damage at tDNAs occurs during DNA replication ( Fig. 5 ). However, Pif1, whose abundance is highest at the end of the S-phase [55] , may also promote R-loop and/or protein removal at tDNAs prior to chromosome condensation and mitosis. 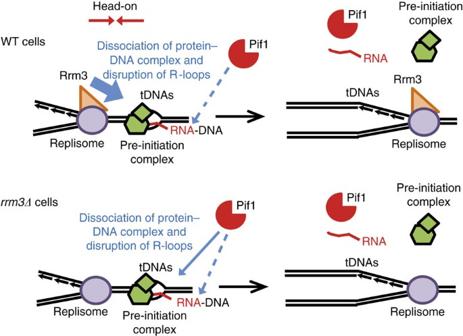Figure 5: Model for Pif1 and Rrm3 function at tDNAs. During replication, Rrm3 plays the main role (thick blue arrow) in promoting replication fork progression and maintaining genome integrity at tDNAs by displacing both the RNA Pol III pre-initiation complex, which impedes fork progression, and R-loops, which cause DNA damage. Pif1 provides a backup for Rrm3 in both R-loop removal (dashed blue arrow) and protein displacement (thin blue arrow) at replicating tDNAs. Figure 5: Model for Pif1 and Rrm3 function at tDNAs. During replication, Rrm3 plays the main role (thick blue arrow) in promoting replication fork progression and maintaining genome integrity at tDNAs by displacing both the RNA Pol III pre-initiation complex, which impedes fork progression, and R-loops, which cause DNA damage. Pif1 provides a backup for Rrm3 in both R-loop removal (dashed blue arrow) and protein displacement (thin blue arrow) at replicating tDNAs. Full size image In conclusion, our study links R-loops at tDNAs to DNA damage and uncovers roles for Pif1 family helicases in suppressing this damage. Pif1 family helicases are found in almost all eukaryotes and are highly conserved [3] . Pfh1, the fission yeast Pif1 family helicase, is critical for promoting fork progression and suppressing DNA damage at tDNAs, 5S genes and highly transcribed RNA Pol II genes [56] , and it unwinds RNA–DNA hybrids efficiently in vitro (M. Wallgren and N. Sabouri, personal communication). Hence, Pfh1 is also likely to suppress R-loop caused DNA damage. Eukaryotic genomes have a large number of highly transcribed RNA Pol III genes (e.g., ∼ 500 tDNAs and 400 5S rRNA genes in the haploid human genome) [57] , [58] . R-loops at RNA Pol III genes may be a heretofore unappreciated source of DNA damage that would occur in all cell types. There is increasing evidence that mutations in human genes that inhibit R-loop disassembly at RNA Pol II genes are associated with human disease [11] , [59] , [60] , [61] , [62] . If human PIF1, like its fungal relatives, resolves R-loops at RNA Pol III genes, this activity may be relevant to human health. Yeast strains All yeast strains were derivatives of YPH499 (ref. 63). Yeast strains, plasmids and primers are listed in Supplementary Tables 9–12 . Gene disruptions and epitope tagging of proteins were confirmed by PCR, DNA sequencing, Southern blotting, western blotting and/or phenotypic analysis. Chromatin immunoprecipitation and quantitative PCR Epitope tagging of proteins for ChIP experiments was done as previously described [7] , [8] . Briefly, cells were grown overnight and harvested at an OD 660 of 0.5. Cells were crosslinked with 1% formaldehyde for 10 min. Chromatin purification was done as described [7] , [8] , except that DNA was sheared to an average size of 300 bps using E220 evolution Focused-ultrasonicator (Covaris, MA, USA). Anti-MYC monoclonal antibody (Clontech #631206) was diluted to 0.02 μg μl −1 and coupled to 80 μl of Dynabeads protein G (ThermoFisher #10004D). After crosslinking reversal and DNA purification, the immunoprecipitated and input DNA were analysed by qPCR using iQ SYBR Green Supermix (Bio-Rad #170-8882) and CFX96 real-time system (Bio-Rad). Samples were analysed in triplicates on three independent ChIP samples for each genotype. Strains and primers are listed in Supplementary Table 9 . Wild-type YPH499 cells without an Myc-tagged protein were used as a control. Western blotting Ten microlitres of cell extract from the input samples from ChIP experiments was analysed by western blotting. Briefly, cell extract was mixed with SDS–polyacrylamide gel electrophoresis sample buffer, boiled for 10 min and pelleted. Samples were loaded onto 15% (37.5:1 polyacrylamide:bis-acrylamide) SDS–polyacrylamide gel electrophoresis gels and run at 20 V cm −1 . The proteins were transferred to a nitrocellulose membrane at 4 °C and blocked with 5% non-fat milk in TBST at room temperature using standard protocols. The blot was probed with an anti-MYC monoclonal antibody (Clontech #631206), which was diluted to 1:500 and visualized with an horseradish peroxidase -conjugated secondary antibody and ECL detection reagents (GE Healthcare). The loading control was obtained by reprobing the blot with an anti-alpha-tubulin antibody (Sigma #T6074) diluted 1:4,000. The quantification of protein levels is the mean of three different western blots. The full western blots are presented in Supplementary Fig. 7 . DR recombination assay DR recombination assays were done in yeast strain yBL3100, a derivative of YPH499 in which ADE2 was integrated on chromosome VI between ORF yFR020W and yFR021W. Test sequences ( tDNA ala and tDNA tyr ) from yeast DNA were cloned in both orientations into the pA2DRIV-B vector, which contains URA3 and a portion of ADE2 (ref. 34) ( Fig. 3a ). This vector with and without a tDNA was introduced by transformation into yBL3100 cells. The vectors were targeted into the inserted ADE2 gene in a manner that disrupted ADE2 to generate the DR substrate. Ura3 − Ade2 + recombinants were detected by growth on plates containing 5-FOA and lacking adenine. At least nine cultures from three independent replicates were grown to saturation in the absence of uracil for 2 days at 30 °C. Dilutions (1:10,000,000) were plated onto non-selective plates to determine the number of viable cells; 100–150 μl was plated on selective plates (1 g l −1 5-FOA, no adenine). Plates were incubated for 4–5 days at 30 °C. Recombination frequencies were determined by dividing the number of recombinant cells by the number of viable cells. The mean recombination frequencies and standard deviations (s.d.) are from at least three independent technical and biological replicates per strain ( Supplementary Table 5 ). P -values are calculated and presented in Supplementary Table 6 . To observe the effects of R-loops at tDNAs, DR strains were transformed with the p424 GAL1 vector or with the same vector containing Rnh1 expressed [47] from the galactose-inducible GAL1 promoter ( Supplementary Table 11 , bottom). Two-millilitre cultures of each DR strain were grown overnight at 30 °C in medium containing 2% raffinose and no tryptophan (selects for plasmid) or uracil (selects against recombinants). Each culture were diluted to OD 660 of ∼ 0.2 and grown in 2% galactose medium lacking both tryptophan and uracil for 24 h at 30 °C. Cells were pelleted and then resuspended to an OD 660 of ∼ 0.25 in medium containing 2% galactose and no tryptophan and then grown for two generations at 30 °C. Dilutions were plated onto non-selective plates to determine the number of viable cells and selective plates (1 g l −1 5-FOA, no adenine and no tryptophan) and grown for 4–5 days at 30 °C to determine the number of recombinants. Recombination frequencies were determined by dividing the number of recombinant cells by the number of viable cells. The means of recombination frequency and standard deviations were obtained from at least three independent technical and biological replicates per strain ( Supplementary Table 7 ). P -values are calculated and presented in Supplementary Table 8 . GCR assay This GCR assay, which detects GCR events in the ∼ 45 terminal kb of the left arm of chromosome V, was developed in Richard Kolodner’s lab [35] . GCR events are selected by the simultaneous loss of URA3 and CAN1 that are present naturally ( CAN1 ) or by insertion ( URA3 ) ( Fig. 3d ). The parent GCR strain was modified by inserting tDNA ala between PRB1 and CIN8 . In a control experiment, we inserted TRP1 instead of a tDNA into the test interval. Insertion of TRP1 did not have a significant effect on GCR rates ( Supplementary Fig. 8 ). To obtain GCR rates, sets of five 5-ml cultures of each S. cerevisiae GCR strain ( Supplementary Table 11 top) were grown to saturation in YEPD medium at 30 °C for 2 days. Dilutions were plated onto non-selective plates and incubated at room temperature for 4 days to determine the number of viable cells. Cells were pelleted, resuspended in sterile water, plated on 5-FOA (1 g l −1 ) plus canavanine sulphate (60 mg l −1 ) minus uracil and arginine, and incubated at 30 °C for 4–5 days to determine the number of GCR events. GCR rates were calculated using FALCOR and the MMS maximum likelihood method [64] . Rates are the mean±s.d. of ≥3 independent experiments per strain ( Supplementary Table 1 ). P -values are calculated and presented in Supplementary Table 2 . To observe the effects of RNA-DNA hybrids at tDNAs, GCR strains were transformed with an empty vector or the same vector expressing Rnh1 from the galactose inducible GAL1 promoter as described above ( Supplementary Table 11 bottom). Sets of five 5 ml cultures of each GCR strain were grown to saturation at 30 °C for 4 days in medium containing 2% galactose and no tryptophan to maintain the vector. Each culture was plated on complete plates lacking tryptophan to determine the number of viable cells and on medium lacking tryptophan, uracil and arginine supplemented with 5-FOA (1 g l −1 ) and canavanine sulphate (60 mg l −1 ) to select for cells that lost expression of URA3 and CAN1 . The rates are the mean±s.d. of ≥3 independent experiments per strain ( Supplementary Table 3 ). P -values are calculated and presented in Supplementary Table 4 . 2D agarose gel electrophoresis Replication intermediates were analysed by standard 2D agarose gel electrophoresis techniques performed on total genomic DNA isolated from asynchronous cells [65] . Cells were collected in early log phase at OD 660 of ∼ 0.6. Collected DNA was restriction enzyme digested (see figure legends for specific enzyme). In the first dimension, DNA was separated in 0.4% agarose at room temperature for 18–22 h depending on the size of the desired DNA fragment at 2.0 V cm −1 . The second dimension was run for 13–15 h in 1.1% agarose containing ethidium bromide (0.3 μg ml −1 ) at 4.4 V cm −1 at 4 °C. Gels were analysed by Southern blotting using 32 P-labelled probes. The extent of pausing was obtained using a typhoon scanner in the following manner. The 32 P signal corresponding to the pause was obtained using ImageQuant TL software by first obtaining the overall intensity of the pause ( Supplementary Fig. 1 , label A 1 ). Background signal was obtained by measuring intensity from an equal portion of the blot at a location that was offset from the pause site ( Supplementary Fig. 1 , label A 2 ) and subtracted from the overall pause signal. The same steps were taken for a portion of the ascending y-arc ( Supplementary Fig. 1 , labels B 1 and B 2 ). The intensity of the pause for a given blot was normalized to replicating molecules by calculating the [pause/y-arc] ratio, [(A 1 -A 2 )/(B 1 -B 2 )]. Quantification of pausing was done in two independent biological replicates and was normalized to the WT pause signal to obtain fold increase relative to WT for each strain. This quantitation method is different from that used previously [5] , where extent of pausing was determined by dividing the 32 P signal in the pause by the signal in the 1N spot using a Molecular Dynamics 400A PhosphorImager. Data availability All data generated or analysed during this study are included in this published article and its Supplementary Files and are available from the corresponding author upon request. How to cite this article: Tran, P. L. T. et al . PIF1 family DNA helicases suppress R-loop mediated genome instability at tRNA genes. Nat. Commun. 8, 15025 doi: 10.1038/ncomms15025 (2017). Publisher’s note: Springer Nature remains neutral with regard to jurisdictional claims in published maps and institutional affiliations.